Plasmonic photosynthesis of C1–C3hydrocarbons from carbon dioxide assisted by an ionic liquid 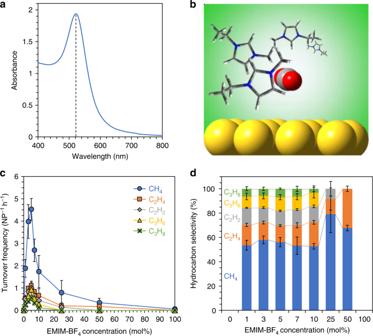Fig. 1 Ionic-liquid-promoted CO2reduction to C1–C3hydrocarbons using a plasmonic Au nanoparticle (NP) photocatalyst.aUV−vis extinction spectrum of a colloid of the Au NPs used for preparation of the photocatalyst film. The spectrum exhibits a localized surface plasmon resonance (LSPR) band centered around 520 nm, as indicated by the dotted line.bScheme for CO2conversion on plasmon-excited Au NPs promoted by an ionic liquid, EMIM-BF4. A continuous-wave (CW) laser of a wavelength of 532 nm and intensity of 1 W cm–2was used as the light source for photoexcitation of Au NPs. EMIM-BF4stabilizes CO2and resulting adsorbates/intermediates on the photoexcited Au surface.cTurnover frequencies of hydrocarbon products formed in the CO2RR plotted as a function of the EMIM-BF4concentration (mol%). The CO2conversion activity peaks at 5 mol% of EMIM-BF4.dHydrocarbon product selectivity as a function of EMIM-BF4concentration (mol%). Each data point incanddis the average of results from three identical trials and the error bar represents the SD of these measurements Photochemical conversion of CO 2 into fuels has promise as a strategy for storage of intermittent solar energy in the form of chemical bonds. However, higher-energy-value hydrocarbons are rarely produced by this strategy, because of kinetic challenges. Here we demonstrate a strategy for green-light-driven synthesis of C 1 –C 3 hydrocarbons from CO 2 and H 2 O. In this approach, plasmonic excitation of Au nanoparticles produces a charge-rich environment at the nanoparticle/solution interface conducive for CO 2 activation, while an ionic liquid stabilizes charged intermediates formed at this interface, facilitating multi-step reduction and C–C coupling. Methane, ethylene, acetylene, propane, and propene are photosynthesized with a C 2+ selectivity of ~50% under the most optimal conditions. Hydrocarbon turnover exhibits a volcano relationship as a function of the ionic liquid concentration, the kinetic analysis of which coupled with density functional theory simulations provides mechanistic insights into the synergy between plasmonic excitation and the ionic liquid. Carbon dioxide (CO 2 ) fixation is recognized to be a much-needed component of a carbon-neutral energy strategy [1] , [2] , [3] , [4] . Although CO 2 is relatively unreactive, various catalytic processes triggered by heat (thermochemical) [5] , [6] , [7] , [8] , electricity (electrochemical) [9] , [10] , [11] , [12] , [13] , [14] , [15] , [16] , [17] , and light (photochemical) [18] , [19] , [20] , [21] , [22] , [23] , [24] , [25] , [26] , [27] , [28] are being explored for activating CO 2 and recycling it back to valuable petrochemicals. Sunlight-driven conversion of CO 2 to fuels is particularly attractive as a means to store intermittent solar energy in the form of C–C and C–H bonds. Semiconductor and metal-catalyzed photoelectrolytic reduction of CO 2 has shown promise; however, these processes have often required ultraviolet (UV) light and/or considerable electrical energy input, or they do not favor energy-rich hydrocarbon products. Longer-chain hydrocarbons possess higher energy densities. Moreover, hydrocarbons in the liquid state are easier to transport [29] , [30] . However, the formation of longer-chain hydrocarbons from CO 2 requires multiple electron (e – ) and proton (H + ) transfer steps, as well as C–C bond formation [9] , [31] , [32] , which pose major kinetic bottlenecks. Here we demonstrate a visible-light-driven route for the conversion of CO 2 and H 2 O into C 1 –C 3 hydrocarbons. The scheme does not involve the application of an electrochemical potential, UV light, high temperatures, hydrogen gas, or a sacrificial agent. It uses green light as the sole energy input and driving agent. The strategy employs plasmonic Au nanoparticles (NPs) of a pseudospherical shape and an average diameter of ~12 nm, as characterized previously [28] . Au NPs are known from electrochemical studies [33] to activate CO 2 . The choice of Au NPs was further driven by the relative chemical stability of Au against bulk oxidation and photocorrosion; the other two common plasmonic metals, Ag and Cu, while electrocatalytically active for CO 2 reduction, are prone to oxidation in air, water, and/or light excitation. The Au NPs possess a strong localized surface plasmon resonance (LSPR) band centered around 520 nm (Fig. 1a ), which enables strong, resonant absorption of green light. The LSPR excitation of the NPs yields energetic electron–hole (e – –h + ) carriers via Landau damping. These e – –h + carriers were shown in recent studies to drive redox conversions [28] , [34] , [35] , [36] , especially the conversion of CO 2 to methane and ethane under blue–green light [28] . However, in this past demonstration, isopropanol was used as a sacrificial h + scavenger to facilitate e – –h + pair separation; otherwise, unproductive e – –h + recombination dominated. Thus, isopropanol served as the H + source in this CO 2 reduction scheme, which posed a major limitation for net energy storage. Fig. 1 Ionic-liquid-promoted CO 2 reduction to C 1 –C 3 hydrocarbons using a plasmonic Au nanoparticle (NP) photocatalyst. a UV−vis extinction spectrum of a colloid of the Au NPs used for preparation of the photocatalyst film. The spectrum exhibits a localized surface plasmon resonance (LSPR) band centered around 520 nm, as indicated by the dotted line. b Scheme for CO 2 conversion on plasmon-excited Au NPs promoted by an ionic liquid, EMIM-BF 4 . A continuous-wave (CW) laser of a wavelength of 532 nm and intensity of 1 W cm –2 was used as the light source for photoexcitation of Au NPs. EMIM-BF 4 stabilizes CO 2 and resulting adsorbates/intermediates on the photoexcited Au surface. c Turnover frequencies of hydrocarbon products formed in the CO 2 RR plotted as a function of the EMIM-BF 4 concentration (mol%). The CO 2 conversion activity peaks at 5 mol% of EMIM-BF 4 . d Hydrocarbon product selectivity as a function of EMIM-BF 4 concentration (mol%). Each data point in c and d is the average of results from three identical trials and the error bar represents the SD of these measurements Full size image The present strategy overcomes this drawback and uses water as the H + source and does not require a sacrificial h + scavenger, thus constituting a truly fuel-forming reaction. The enhanced reactivity was enabled by the use of an ionic liquid (IL) medium, specifically comprised 1-ethyl-3-methylimidazolium tetrafluoroborate (EMIM-BF 4 ). Our choice was motivated by examples from electrocatalytic CO 2 reduction reaction (CO 2 RR) where the EMIM-BF 4 electrolyte, owing to its highly ionic character, stabilizes the high-energy CO 2 • − radical anion intermediate formed in the reaction and decreases the overpotential needed for CO 2 RR [37] , [38] , [39] , [40] , [41] , [42] . In addition, EMIM-BF 4 has a wide electrochemical window and high thermal stability [43] , [44] . In our photocatalytic scheme, the EMIM-BF 4 , as we find from kinetic analysis and density functional theory (DFT) simulations, promotes e – transfer at the interface of the photoexcited Au NP and adsorbed CO 2 (Fig. 1b ), obviating the need for a h + scavenger or applied potential for e – –h + separation. IL-mediated plasmonic CO 2 reduction The photocatalyst had the form of a substrate-supported film of Au NPs immersed in an aqueous solution of EMIM-BF 4 saturated with CO 2 and contained inside a glass reactor ( Supplementary Methods ). The light excitation source comprised a continuous-wave (CW) laser of a wavelength of 532 nm light and an intensity of 1 W cm −2 . Under CW excitation, the steady-state temperature of the reaction medium got moderately elevated to ~48 °C. Hydrocarbon products collected in the reactor headspace were measured (Supplementary Figs. 1 − 11 ) using a gas chromatograph (GC) equipped with a flame ionization detector. The EMIM-BF 4 concentration was varied from 0 to 100 mol%, to find optimal conditions for CO 2 RR. In 1–10 mol% EMIM-BF 4 , the products of plasmon-excitation-driven CO 2 RR were found to be C 1 (CH 4 ), C 2 (C 2 H 4 and C 2 H 2 ), and highly reduced C 3 (C 3 H 6 and C 3 H 8 ) hydrocarbons (Fig. 1c, d and Supplementary Note 1 ). This product profile is quite striking when one considers that the major product in electrochemical CO 2 RR is carbon monoxide (CO) formed by 2e – –2H + reduction of CO 2 (refs. [13] , [14] , [15] , [16] , [17] ). On the other hand, propane (C 3 H 8 ), formed in our scheme, requires an overall 20e – –20 H + reduction and coupling of three CO 2 molecules. Such generation of C 3 hydrocarbons by artificial photosynthesis is challenging and therefore rare. The CO 2 RR activity depends on the IL concentration (Fig. 1c ). In pure water the activity was nil, whereas in 1 mol% EMIM-BF 4 solution the generation of C 1 , C 2 , and C 3 hydrocarbons was observed. The CO 2 RR activity, as quantified by turnover frequencies (TOFs) of the hydrocarbon products, increased dramatically with an increase in the EMIM-BF 4 concentration. The highest activity was found at 5 mol% EMIM-BF 4 . Increasing the EMIM-BF 4 concentration further resulted in a sharp drop in the CO 2 RR activity. In 100 mol% EMIM-BF 4 solution, the activity was nil, similar to that in pure water. Thus, the CO 2 RR activity exhibits a volcano relationship as a function of the EMIM-BF 4 concentration (Fig. 1c ). At all EMIM-BF 4 concentrations, where C 1 , C 2 , and C 3 hydrocarbons were produced, the product selectivity was found to follow the order: C 1 > C 2 > C 3 . The selectivity for C 2+ production is ~50% in 1−10 mol% EMIM-BF 4 solution (Fig. 1d ). Non-hydrocarbon products were also characterized by a GC equipped with a thermal conductivity detector (TCD) (Supplementary Figs. 12 – 15 ). Considerable hydrogen (H 2 ) production was measured (Supplementary Fig. 12 ), the TOF of which was 138.2 NP − 1 h −1 in 5 mol% EMIM-BF 4 solution, the IL concentration where CO 2 RR activity is the highest. The H 2 likely originates from the competing reduction of H + in the reaction medium (Supplementary Eq. (6 ) ). In the GC-TCD measurements, there were no detection of CO (Supplementary Fig. 15 ), otherwise known to be a major product in electrocatalytic CO 2 RR on Au (refs. [13] , [14] , [15] , [16] , [17] ). Of the possible oxidation products, there was no measurable production of O 2 (see Supplementary Information ). H 2 O 2 was detected (Supplementary Figs. 16 – 18 ) by the fluorogenic test employing a amplex red and horseradish peroxidase reagent [45] . Thus, the oxidation of H 2 O to H 2 O 2 and H + (2H 2 O → H 2 O 2 + 2H + + 2e − ) is the likely oxidation half-reaction that consumes the photogenerated h + . Control studies were performed, one without Au NPs, another without light, and a third without CO 2 . The conditions were otherwise maintained the same as those in the photoreaction tests and a 5 mol% EMIM-BF 4 solution, found to be most optimal in the photoreaction tests, was employed. The control studies showed that the absence of any one of the components Au NPs, green light illumination, or CO 2 resulted in nil hydrocarbon production, despite the use of 5 mol% EMIM-BF 4 solution (Supplementary Fig. 19a–c ). Thus, it is confirmed that the hydrocarbon production originates from green-light-driven CO 2 reduction on Au NPs. The control study without light excitation was performed at an elevated temperature of 50 °C so as to mimic the steady-state bulk solution temperature of the reaction mixture in the photoreaction tests. The lack of CO 2 RR activity in this dark control study demonstrates that the CO 2 RR activity in the photoreaction tests does not originate from simply a photothermal effect of the light excitation. Rather a photoredox process facilitated by the Au NPs and the IL is responsible for the conversion of CO 2 to hydrocarbons. The plasmonic catalyst also exhibited stability and recyclability under the photoreaction conditions and IL media subjected on the catalyst. We tested the same substrate-supported Au NP film immersed in 5 mol% EMIM-BF 4 over multiple cycles, each consisting of a 10 h photoreaction. The CO 2 RR activity and product selectivity, as determined from the TOFs of the hydrocarbon products, was maintained over the course of this multi-cycle test (Supplementary Fig. 20 ). As the NP film or EMIM-BF 4 solution were not replenished between cycles, the maintenance of CO 2 RR activity over multiple cycles suggests that Au and EMIM-BF 4 were not consumed, at any discernible levels, in the photoredox reaction. The origin of products Given the hydrocarbon profile of the product mixture, it was necessary to go beyond the control studies described above and confirm more directly that CO 2 , rather than carbon contamination or photolysis of the EMIM-BF 4 , was the source of the hydrocarbon products. For this confirmation, 13 C isotope labeling was employed (Fig. 2 and Supplementary Figs. 21 and 22 ). In this labeling study, 13 CO 2 was employed as the reactant instead of 12 CO 2 , whereas all other conditions were kept the same as those in other photoreaction tests. GC-mass spectrometry (GC-MS) was used for identification of the hydrocarbon products generated in the photoreaction (Fig. 2a ). The GC-MS analysis confirmed the presence of 13 CH 4 (Fig. 2b ) and 13 C 2 H 2 (Fig. 2c ), manifested by their characteristic mass fragmentation patterns, shifted to higher m/z compared with reference fragmentation patterns of 12 CH 4 and 12 C 2 H 2 , respectively. Thus, isotope labeling confirms CO 2 to be the origin of hydrocarbon products. Fig. 2 13 CO 2 isotopolog confirmation of CO 2 RR. a Total ion chromatogram (TIC) of the gaseous products from a 240 h long Au NP-photocatalyzed 13 CO 2 RR in 5 mol% EMIM-BF 4 solution under CW irradiation of 532 nm light (1 W cm –2 ). Peaks in the TIC appearing at retention times of 4.6 min and 8.2 min correspond to 13 CH 4 and 13 C 2 H 2 . The basis for this assignment is provided in Supplementary Fig. 22 . b Mass fragmentation pattern (red bars) acquired at a retention time of 4.6 min of the TIC shown in a . For comparison, a reference fragmentation pattern (gray bars) of 12 CH 4 from the National Institute of Standards and Technology (NIST) Chemistry WebBook is shown. Fragments at m/z = 14 and 18 in the experimental pattern were suppressed to remove the mass peaks contributed by N 2 and moisture, respectively. c Mass fragmentation pattern (blue bars) acquired at a retention time of 8.2 min of the TIC shown in a . For comparison, a reference fragmentation pattern (gray bars) of 12 C 2 H 2 from the NIST Chemistry WebBook is shown. The fragment at m/z = 28 in the experimental pattern has relatively high abundance as compared with that of the reference fragmentation pattern due to the contribution of N 2 from the atmosphere. Relative abundances in b and c were obtained from the measured abundances shown in Supplementary Fig. 21a, b , respectively. It is noteworthy that 13 C 2 H 4 was not resolved by GC-MS due to the likely overlap of the 13 C 2 H 4 peak with the broad, intense 13 CO 2 peak in the TIC (Supplementary Fig. 22b ) Full size image The role of the IL We attempted to gain a mechanistic understanding of this catalytic scheme focusing on the question of how the IL promotes CO 2 RR activity. It was observed that the presence of EMIM-BF 4 in the aqueous medium results in a considerably acidic pH (Supplementary Fig. 23 ): the 5 mol% EMIM-BF 4 solution has a pH of 2.95. To determine whether this acidity is responsible for the enhanced CO 2 RR activity in a EMIM-BF 4 solution, we performed a photoreaction in deionized water containing no EMIM-BF 4 but with a pH of 2.93 achieved using acid (Supplementary Fig. 19d ). All other conditions were kept the same as in the photoreactions in EMIM-BF 4 solutions. In this EMIM-BF 4 -free photoreaction, no products were observed, which demonstrated that the high acidity or H + concentration, [H + ], of the EMIM-BF 4 -containing medium is not the sole cause of the enhanced CO 2 RR activity. EMIM-BF 4 plays other role(s). It is possible, in principle, for EMIM-BF 4 , instead of H 2 O, to serve as the h + acceptor; however, if this were the case, then the CO 2 RR activity would have been enhanced at higher EMIM-BF 4 concentrations, in line with a study of a different plasmon excitation-catalyzed redox reaction [36] . Instead, we observed peak activity at a EMIM-BF 4 concentration of 5 mol%, above which the activity drops steeply reaching nil in pure EMIM-BF 4 wherein H 2 O is not available. We hypothesized that the strongly ionic character of EMIM-BF 4 plays a role in the activation of CO 2 , which is otherwise fairly redox inactive. CO 2 , however, is highly polarizable, as indicated by its quadrupole moment of −4.3 D Å (ref. 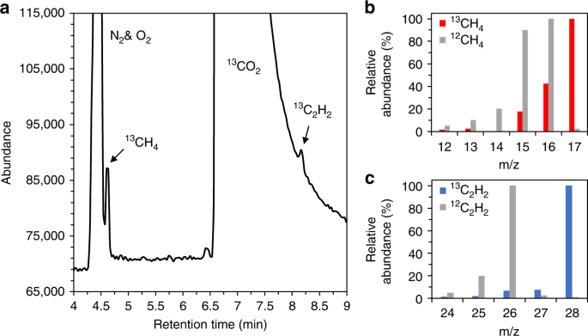Fig. 2 13CO2isotopolog confirmation of CO2RR.aTotal ion chromatogram (TIC) of the gaseous products from a 240 h long Au NP-photocatalyzed13CO2RR in 5 mol% EMIM-BF4solution under CW irradiation of 532 nm light (1 W cm–2). Peaks in the TIC appearing at retention times of 4.6 min and 8.2 min correspond to13CH4and13C2H2. The basis for this assignment is provided in Supplementary Fig.22.bMass fragmentation pattern (red bars) acquired at a retention time of 4.6 min of the TIC shown ina. For comparison, a reference fragmentation pattern (gray bars) of12CH4from the National Institute of Standards and Technology (NIST) Chemistry WebBook is shown. Fragments at m/z = 14 and 18 in the experimental pattern were suppressed to remove the mass peaks contributed by N2and moisture, respectively.cMass fragmentation pattern (blue bars) acquired at a retention time of 8.2 min of the TIC shown ina. For comparison, a reference fragmentation pattern (gray bars) of12C2H2from the NIST Chemistry WebBook is shown. The fragment at m/z = 28 in the experimental pattern has relatively high abundance as compared with that of the reference fragmentation pattern due to the contribution of N2from the atmosphere. Relative abundances inbandcwere obtained from the measured abundances shown in Supplementary Fig.21a, b, respectively. It is noteworthy that13C2H4was not resolved by GC-MS due to the likely overlap of the13C2H4peak with the broad, intense13CO2peak in the TIC (Supplementary Fig.22b) [46] ). The interaction of EMIM-BF 4 and CO 2 was simulated by DFT. A past study suggests that CO 2 can undergo complexation with the N -heterocyclic carbene, EMIM * , formed from EMIM + by H + loss [42] . We investigated using DFT the structure of such a [EMIM*-CO 2 ] complex (Fig. 3a ). The complex exhibits binding between the C atom of the CO 2 and the C 2 atom of the imidazole ring with an energy of intermolecular interaction, E m-m , of −0.36 eV. This interaction is stronger than, for instance, the interaction of an H 2 O molecule and CO 2 (Fig. 3b ). Unlike the latter case, complexation with EMIM * leads to considerable restructuring of the CO 2 moiety. The CO 2 moiety adopts a bent configuration with an O=C=O angle of 133.7° and C=O bonds lengthened to 1.24 Å. In fact, the geometry of the CO 2 moiety in the complex closely mirrors that of the CO 2 •− anion radical, which has a bond angle of 137.8° and bond length of 1.23 Å (Supplementary Fig. 24 ). Moreover, from Mulliken charge partitioning analysis (Supplementary Fig. 25 ), the CO 2 moiety in the [EMIM*-CO 2 ] complex is found to have a net charge of −0.73, which indicates its partial anionic character. Fig. 3 The role of the ionic liquid in Au NP-photocatalyzed CO 2 RR. a , b DFT-optimized geometries of [EMIM*-CO 2 ] ( a ) and [H 2 O-CO 2 ] ( b ) complexes. C, H, O, and N atoms are depicted by gray, white, red, and blue spheres, respectively. Key bond lengths, bond angles, and the energy of intermolecular interaction, E m-m , are indicated for each of the complexes. c – e DFT-computed free energy cost, ∆ G , of formation of the 1e − adduct of CO 2 ( c ), 1e − adduct of [EMIM*-CO 2 ] ( d ), and 1e − adduct of CO 2 in the presence of EMIM + ( e ). 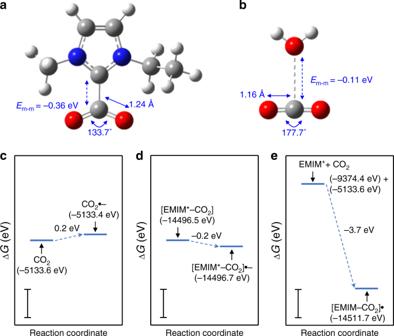Fig. 3 The role of the ionic liquid in Au NP-photocatalyzed CO2RR.a,bDFT-optimized geometries of [EMIM*-CO2] (a) and [H2O-CO2] (b) complexes. C, H, O, and N atoms are depicted by gray, white, red, and blue spheres, respectively. Key bond lengths, bond angles, and the energy of intermolecular interaction,Em-m, are indicated for each of the complexes.c–eDFT-computed free energy cost, ∆G, of formation of the 1e−adduct of CO2(c), 1e−adduct of [EMIM*-CO2] (d), and 1e−adduct of CO2in the presence of EMIM+(e). In the latter case, the 1e−adduct of CO2, CO2•−, is stabilized by complexation with EMIM+as described by the net process: EMIM++ CO2+ e−→ [EMIM-CO2]•. Inc–e, the free energy of each species is indicated in parentheses. Scale bars are 1 eV in length 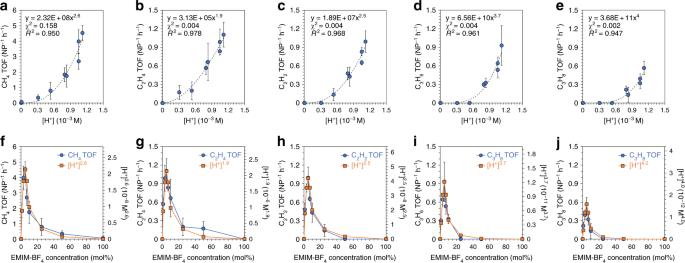Fig. 4 Empirical kinetic model for the CO2RR.a–eFor each of the hydrocarbon products, the TOF is plotted as a function of the H+concentration, [H+], which serves as a proxy for the concentration of the [EMIM*-CO2] complex. A fit to a power-law functiony=axn(dashed line) yields the fit parametern, which represents the apparent reaction order in [H+]. The best-fit equation is indicated for each plot along with the values ofχ2andR2, which serve as metrics of the goodness-of-fit.f–jFor each hydrocarbon product, the TOF plotted as a function of the EMIM-BF4concentration follows a similar trend as the [H+]n, wherenis the corresponding reaction order obtained from the plots ina–e. Each data point ina–jis the average of results from three identical trials and the error bar represents the SD of these measurements In the latter case, the 1e − adduct of CO 2 , CO 2 •− , is stabilized by complexation with EMIM + as described by the net process: EMIM + + CO 2 + e − → [EMIM-CO 2 ] • . In c – e , the free energy of each species is indicated in parentheses. Scale bars are 1 eV in length Full size image It is known that the energetic cost of the drastic structural reorganization from linear CO 2 to the bent CO 2 •− anion radical poses a major barrier for e − acceptance by CO 2 (refs. [37] , [38] , [39] , [40] , [41] , [42] ). However, our DFT calculations show that in its complex with EMIM*, the CO 2 moiety is structurally pre-configured for e − acceptance. Consistent with this finding, 1e – addition to [EMIM*-CO 2 ] is much more favorable as compared with 1e − addition to CO 2 (Fig. 3c, d ). Thus, it appears that EMIM-BF 4 can promote the transfer of photogenerated e – from the Au NP to adsorbed CO 2 , which is otherwise a major kinetic bottleneck in the photocatalytic reduction process. Furthermore, it is plausible that the CO 2 •− anion radical formed on the Au surface by photo-initiated e – transfer process has an enhanced lifetime due to solvation or complexation by EMIM + (Fig. 3e ). A longer lifetime of this reactive intermediate would increase the probability of C–C coupling between the intermediates. Empirical kinetic model Although the DFT computations provide insight into the central role of EMIM-BF 4 in CO 2 activation, the volcano-type dependence of the CO 2 RR activity on the IL concentration deserves an explanation. From the hydrolysis of EMIM-BF 4 known from past studies [47] , [48] , [49] , [50] : 
    EMIM-BF_4 + xH_2O→EMIM^ + + [ BF_4-x( OH)_x]^- + xHF
 (1) where x = 1–4 and the complexation of CO 2 with EMIM + predicted in DFT simulations: 
    EMIM^ + + CO_2 →[ EMIM^ ∗-CO_2] + H^ +
 (2) we postulate a rate determining step in the reaction of CO 2 and H 2 O: 
    EMIM-BF_4 + CO_2 + xH_2O→[ EMIM^∗-CO_2] 
     + [ BF_4-x( OH)_x]^- + ( x + 1)H^ + + xF^-
 (3) From this reaction equation, the concentration of the activated CO 2 complex, [EMIM*-CO 2 ], is expected to be directly proportional to [H + ] x +1 . Therefore, the [H + ] determined from the measured pH of the EMIM-BF 4 solution (Supplementary Fig. 23 ) serves as a proxy for the concentration of [EMIM*-CO 2 ], based on which the [EMIM*-CO 2 ] concentration is expected to be the highest in the EMIM-BF 4 concentration range around 5 mol%. The higher the concentration of the activated [EMIM*-CO 2 ] complex, the greater is the rate of CO 2 conversion and also the higher the likelihood of C–C coupling required for C 2+ production. Therefore, both the overall activity and the selectivity in favor of C 2+ products are favorable in the 3–7 mol% EMIM-BF 4 range, with the most optimal performance achieved at 5 mol% EMIM-BF 4 . On the other hand, the activated complex has zero concentration in pure water on one extreme and in pure EMIM-BF 4 on the other extreme, which explains the nil turnover at these conditions. An additional reason for the drop in activity at higher EMIM-BF 4 concentrations may be that the adsorption of BF 4 – to the Au NP surface (Supplementary Fig. 26 ) dominates at these concentrations to such an extent that the adsorption of CO 2 and/or [EMIM*-CO 2 ] to the Au surface is largely inhibited and so is the e − transfer to CO 2 . The CO 2 RR activity depends on the concentration of this activated complex to a high reaction order. This is best exemplified by the plots of TOF for each hydrocarbon as a function of the [H + ] (Fig. 4a–e ), which as explained above, serves as a proxy for the concentration of [EMIM*-CO 2 ]. The pseudo-reaction order, n , is found to be 1.9 for C 2 H 4 , 2.5 for C 2 H 2 , 3.7 for C 3 H 6 , and 4.0 for C 3 H 8 . The fit for the CH 4 TOF has a relatively high χ 2 -value, so the n of 2.7 estimated for CH 4 has a lower confidence. In general, the pseudo-reaction order is higher for the longer hydrocarbons, which perhaps captures the need for multiple activated complexes to be available for undergoing coupling to C 2 and C 3 fragments. The high pseudo-reaction order for the C 3 products goes hand-in-hand with an apparent threshold in [H + ] below which the TOF is zero or below the detection limit (Fig. 4d, e ). For each of the hydrocarbon products, the [H + ] raised to the power of the corresponding n follows a volcano trend with respect to the EMIM-BF 4 concentration, mirroring closely the trend in the TOF for that hydrocarbon (Fig. 4f–j ). Fig. 4 Empirical kinetic model for the CO 2 RR. a – e For each of the hydrocarbon products, the TOF is plotted as a function of the H + concentration, [H + ], which serves as a proxy for the concentration of the [EMIM*-CO 2 ] complex. A fit to a power-law function y = ax n (dashed line) yields the fit parameter n , which represents the apparent reaction order in [H + ]. The best-fit equation is indicated for each plot along with the values of χ 2 and R 2 , which serve as metrics of the goodness-of-fit. f – j For each hydrocarbon product, the TOF plotted as a function of the EMIM-BF 4 concentration follows a similar trend as the [H + ] n , where n is the corresponding reaction order obtained from the plots in a – e . Each data point in a – j is the average of results from three identical trials and the error bar represents the SD of these measurements Full size image Thus, we reported the green-light-driven synthesis of C 1 –C 3 hydrocarbons from CO 2 and water on plasmonic Au NPs in an IL medium. The resonant green light absorption of the plasmonic NPs and their ability to sustain electrostatically charged surfaces under resonant CW excitation are at the heart of the observed photoreactivity. The IL plays a synergistic role due to its complexation with the CO 2 , which preconfigures the CO 2 for accepting e – from photoexcited Au NPs. The enhanced reactivity of CO 2 in the presence of the IL obviates the need for an applied potential or a sacrificial scavenger. Although hydrocarbon production yields in the reaction need further optimization, the generation of propane by overall 20e − –20H + reduction and coupling of three CO 2 molecules is both striking and mechanistically rich. The precise intermediates and reaction pathways, including C–C coupling and dehydrogenation steps, which yield each of the hydrocarbons, deserve further elucidation. Beyond CO 2 conversion studied here, ILs may have promise in other photocatalytic schemes where activation of relatively inert substrates and stabilization of high-energy charged intermediates is desirable.